Revealing the molecular structure of single-molecule junctions in different conductance states by fishing-mode tip-enhanced Raman spectroscopy The conductance of single-molecule junctions may be governed by the structure of the molecule in the gap or by the way it bonds with the leads, and the information contained in a Raman spectrum is ideal for examining both. Here we demonstrate that molecule-to-surface bonding may be characterized during electron transport by 'fishing-mode' tip-enhanced Raman spectroscopy (FM-TERS). This technique allows mutually verifiable single-molecule conductance and Raman signals with single-molecule contributions to be acquired simultaneously at room temperature. Density functional theory calculations reveal that the most significant spectral change seen for a gold-4,4′-bipyridine-gold junction results from the deformation of the pyridine ring in contact with the drain electrode at high voltage, and these calculations suggest that a stronger bonding interaction between the molecule and the drain may account for the nonlinear dependence of conductance on bias voltage. FM-TERS will lead to a better understanding of electron-transport processes in molecular junctions. In molecular electronics, individual molecules with unique properties serve as the basic electrical components. This field has attracted increasing interest in recent years [1] , [2] , [3] . Various methods have been established to construct electron-transport junctions, which serve as the main investigative tool in molecular electronics, and to characterize different properties of the active region [4] , [5] , [6] , [7] , [8] , [9] , [10] , [11] . Inelastic electron tunnelling spectroscopy is commonly used to provide structural information about the molecules there, but this technique requires low-temperature and vacuum conditions [12] , [13] , [14] , [15] . Conventional optical spectroscopic methods appear to be the most promising ones with which to examine the correlation between structure and conductance under ambient conditions [16] , [17] , [18] , [19] , [20] , [21] , [22] , [23] ; however, their low spatial resolution has led to interference by molecules other than the one in the junction [1] , [16] . Tip-enhanced Raman spectroscopy (TERS), a type of apertureless scanning near-field optical microscopy, offers a combination of single-molecule sensitivity and ultrahigh spatial resolution [24] , [25] , [26] , [27] , [28] . 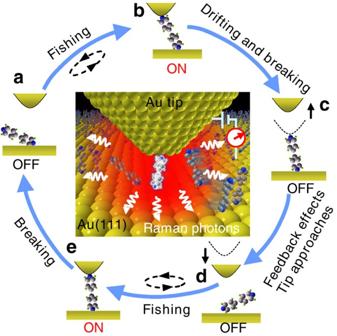Figure 1: Schematic diagram of 'fishing-mode' TERS (FM-TERS). An illustration of the FM-TERS system for simultaneous conductance and TERS measurement of single-molecule junctions. A gold(111) surface is pre-adsorbed with molecules. The distance between the gold tip and the gold(111) surface is then controlled by an STM equipped with a conductance-measuring circuit. The red contour indicates the distribution of electromagnetic field strength between the tip and the substrate. Wavy arrows indicate Raman scattering by the molecules. (a) The tip and the substrate are close enough for a molecular junction to form between them, but the molecule is not yet in contact with the tip. (b) Formation of a molecular junction. (c) Thermal or mechanical drift causes the junction to break. (d) STM feedback takes effect, and it brings the tip back to the previous distance to fish for another molecule. (e) A new junction is formed and the cycle continues. The electromagnetic field-enhancing structure is a gold (or silver) tip, as shown in the centre of Figure 1 . When the tip is brought sufficiently close to the substrate to make contact with molecules adsorbed there, a single-molecule junction will spontaneously form. In general, the tip will be free of molecules except for the one at its apex that forms the junction. Other molecules that are on the substrate and directly underneath the tip will experience the enhanced electromagnetic field to some extent, but the molecule forming the junction will experience the greatest enhancement. Therefore, interference from molecules outside the junction is minimized and spectroscopic information from the junction is predominant. For this reason, TERS would appear to be an ideal tool for studying the structure of a molecular junction. Figure 1: Schematic diagram of 'fishing-mode' TERS (FM-TERS). An illustration of the FM-TERS system for simultaneous conductance and TERS measurement of single-molecule junctions. A gold(111) surface is pre-adsorbed with molecules. The distance between the gold tip and the gold(111) surface is then controlled by an STM equipped with a conductance-measuring circuit. The red contour indicates the distribution of electromagnetic field strength between the tip and the substrate. Wavy arrows indicate Raman scattering by the molecules. ( a ) The tip and the substrate are close enough for a molecular junction to form between them, but the molecule is not yet in contact with the tip. ( b ) Formation of a molecular junction. ( c ) Thermal or mechanical drift causes the junction to break. ( d ) STM feedback takes effect, and it brings the tip back to the previous distance to fish for another molecule. ( e ) A new junction is formed and the cycle continues. Full size image In this work, we introduce 'fishing-mode' scanning tunnelling microscopy (FM-STM), which can be used to obtain high-quality conductance histograms from molecular junctions with great efficiency. We then combine our FM-STM method with TERS to yield 'fishing-mode' TERS (FM-TERS). This can be used to obtain mutually verifiable single-molecule conductance and Raman signals with single-molecule contributions simultaneously at room temperature. We then perform FM-TERS measurements on molecular junctions at different bias voltages, and use theoretical methods to determine structure in the junction at each voltage from the spectral features observed. We are confident that our FM-TERS technique will lead to a better understanding of electron-transport processes in molecular junctions. Principle of FM-STM for measuring single-molecule conductance To obtain a reliable TERS signal while monitoring single-molecule conductance, it is necessary to keep the distance between the tip and the substrate within a suitable range for a considerably long period of time. For this purpose, we developed a new conductance-measuring method. It is based on traditional scanning tunnelling microscopy (STM) but has a critically altered feedback state. Experimentally, we first pre-adsorb a gold(111) surface with molecules. We approach it with the STM tip until an appropriate junction distance is reached ( Fig. 1a ); then we decrease the response of the STM by lowering the proportional gain and the integral gain to about 0.03% of their normal values (we lower it from ~3 to ~0.001). The conductance of the system is continuously recorded. When a molecular junction forms ( Fig. 1b ), current flowing through the STM will increase according to the actual electron-transport properties of the molecule. Under the low-feedback condition, the tip will retract to decrease the current with a rate that is significantly reduced in comparison to the normal feedback-condition rate. As the tip moves away from the gold(111) surface, the junction will break ( Fig. 1c ). Then, the current will drop and the feedback system will force the tip to return to the substrate ( Fig. 1d ) to regain the tunnelling current ( Fig. 1e ). As a result, the tip is confined within a few angstroms of the junction distance, and the instrument can remain stable for several minutes at a time ( Supplementary Fig. S1 ). Thermally driven movement of molecules on the surface will lead to formation and breaking of molecular junctions in the gap with high frequency, and this may be observed as a set of current jumps. The probability of trapping a molecule in the junction and the lifetime of each molecular bridge are both increased by our method in comparison with the STM break-junction and alternating-current modulation methods [6] , [7] . Meanwhile, the low-feedback state remains able to compensate any slow thermal or mechanical instrument drift [7] , in contrast to the feedback-disabled method [9] , [29] . These two advantages allow conductance to be measured continuously over a long period of time with minimal instrument drift interference. We call this 'fishing-mode' STM (FM-STM). To demonstrate the reliability and efficiency of FM-STM for measuring single-molecule conductance, we used 1,8-octanedithiol (1,8-ODT) as a probe molecule, an electrochemically etched gold wire as the STM tip, and a gold(111) surface as the substrate [30] . Hundreds of current jumps were easily obtained in a very short period of time (400 ms), with each current jump on the time scale of a fraction of a ms ( Fig. 2a,b ). These current jumps have been ascribed to formation (the ON-conduction state) and breaking (the OFF-conduction state) of molecular junctions [9] , [29] . We performed a statistical analysis on the current jumps and obtained a characteristic histogram for conductance with a modal value of about 5.6×10 −5 G 0 ( Fig. 2c ), where G 0 =2 e 2 / h corresponds to the conductance of gold at single-atom to single-atom point of contact [6] . This value is comparable with the ones obtained using other methods [6] , [7] , [11] , [29] , [31] . 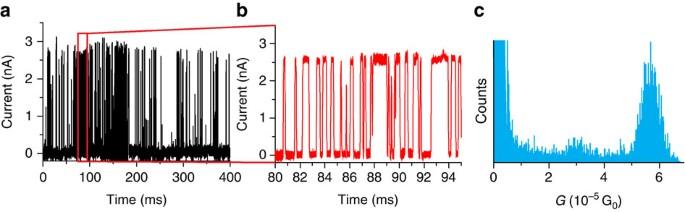Figure 2: Current traces and a conductance histogram obtained by FM-STM for 1,8-ODT. (a) A time-sequence conductance curve for 1,8-ODT in the junction between the gold tip and the gold(111) substrate (bias voltage=600 mV, current set-point=1 nA; the current was background corrected). (b) An expanded view of the region marked with a red outline in (a). (c) The conductance histogram for 1,8-ODT. In addition to demonstrating its reliability, Figure 2 also demonstrates the efficiency of our FM-STM method: it can provide a high-quality conductance histogram in a very short period of time down to half a second (see Supplementary Fig. S2 for the comparison) [31] . Moreover, the low-feedback state employed is sufficient to confine the tip within a few angstroms of the pre-set value during the whole process. This is essential for combination with TERS. Figure 2: Current traces and a conductance histogram obtained by FM-STM for 1,8-ODT. ( a ) A time-sequence conductance curve for 1,8-ODT in the junction between the gold tip and the gold(111) substrate (bias voltage=600 mV, current set-point=1 nA; the current was background corrected). ( b ) An expanded view of the region marked with a red outline in ( a ). ( c ) The conductance histogram for 1,8-ODT. Full size image Simultaneous conductance and TERS measurement We then combined the ability to measure single-molecule conductance by our FM-STM method, with the ability to acquire Raman spectra having single-molecule contributions by TERS. We call this second technique 'fishing-mode' TERS (FM-TERS). We used 4,4′-bipyridine (4bipy), a common probe in both molecular electronics and surface-enhanced Raman scattering (SERS), as the junction-forming molecule [6] , [10] , [17] and we obtained conductance data ( Fig. 3a ) and TERS spectra ( Fig. 3b ) from the gold tip-4bipy-gold(111) junction system at the same time. Again, the key feature of our FM-TERS method is that it allows both of these data types to be acquired from a single-molecule junction simultaneously. An expanded view of the conductance curve (left inset of Fig. 3a ) shows some characteristic current jumps. A statistical analysis of the ON-state conductance values produced a typical conductance histogram with a modal value of (4.0±1.0)×10 −4 G 0 (right inset of Fig. 3a ) [10] , [31] . 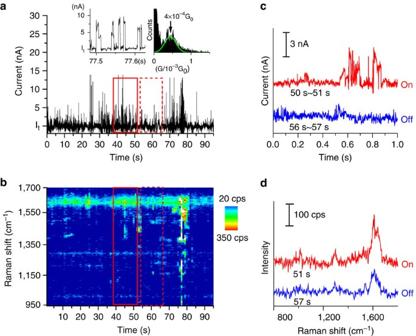Figure 3: Simultaneous conductance and TERS measurement of 4bipy by FM-TERS. (a) Time sequence of conductance for the gold tip-4bipy-gold(111) system (bias voltage=200 mV, tunnelling current (It)=5 nA). Left inset: expanded view of (a); right inset: conductance histogram for the gold tip-4bipy-gold(111) system. (b) Time sequence of 4bipy TERS spectra obtained simultaneously with the conductance data in (a). (c) Selected conductance curves for a 1 s time period. (d) TERS spectra that correspond to the conductance curves in (c). Figure 3: Simultaneous conductance and TERS measurement of 4bipy by FM-TERS. ( a ) Time sequence of conductance for the gold tip-4bipy-gold(111) system (bias voltage=200 mV, tunnelling current ( I t )=5 nA). Left inset: expanded view of ( a ); right inset: conductance histogram for the gold tip-4bipy-gold(111) system. ( b ) Time sequence of 4bipy TERS spectra obtained simultaneously with the conductance data in ( a ). ( c ) Selected conductance curves for a 1 s time period. ( d ) TERS spectra that correspond to the conductance curves in ( c ). Full size image Interestingly, the TERS signal from a period of time with a high probability of ON states shows increased intensities and band widths, and some shifting of band positions (see Fig. 3a and the 'waterfall' plot in Fig. 3b ). To fully understand the correlation between the conductance and the TERS signal, we selected some 1-s conductance curves (with and without current jumps, Fig. 3c ) and their corresponding TERS spectra ( Fig. 3d ) for analysis. Impressively, the TERS signal fluctuates, when the conductance switches between the single-molecule junction (ON) state and the disconnected (OFF) state, indicating that the change in the TERS signal is due to single-molecule events. This result demonstrates the advantage of FM-TERS over the existing correlated conductance and SERS methods [20] , [21] , [32] . Spectral fluctuations are often used as an indicator for single-molecule SERS and TERS, but they may also be caused by degradation of probe molecules in the enhanced electromagnetic field. A simple test has been proposed to distinguish between the different origins of these fluctuations [33] : if the spectral changes are due to nondestructive processes, the signal quality will be maintained over time and spectral averaging will give the far-field ensemble spectrum of the molecule; if, however, the changes are due to photo-induced degradation, spectral averaging will yield a typical carbon spectrum with broad peaks at around 1,350 and 1,580 cm −1 . We therefore used statistics to help us understand the gold tip-4bipy-gold(111) junction system. 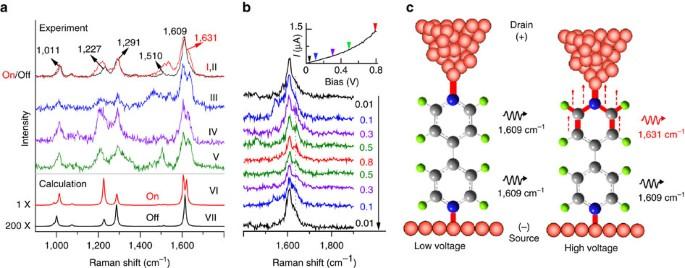Figure 4: FM-TERS of 4bipy in a molecular junction and its bonding configuration. (a) I is an average of all 190 ON-state TERS spectra and II is a typical OFF-state TERS spectrum. Each of III, IV and V correspond to an average of ≥20 ON-state spectra. VI and VII are calculated ON- and OFF-state spectra, respectively. (b) The ν8aband of 4bipy (1609 cm−1) is seen to change with the bias voltage (current set-point=5 nA). Inset: current versus bias curve for 4bipy obtained with a mechanical break-junction setup. (c) This diagram illustrates why 1,609 cm−1band splitting is proportional to the applied bias voltage. When we averaged over all 190 ON-state spectra, we obtained spectrum I (red) in Figure 4a . An OFF-state spectrum is given for comparison (spectrum II, black). We also present three 'typical' spectra, each of which is actually the average of at least 20 ON-state spectra, in the same figure (they are labelled III, IV and V). All five of these spectra display features of 4bipy; however, band intensity, width and position all vary. The absence of carbon bands at 1,350 and 1,580 cm −1 indicates that the spectral fluctuations are not due to photo-induced decomposition of the probe molecule, but reflect dynamic single-molecule events in the junction. We note that because of differences between the way our TERS system and most SERS substrates are prepared, our TERS system is much cleaner initially ( Supplementary Note 1 and Fig. S3 ), and this should help reduce the amount of carbon formed during irradiation. Comparing spectrum I (ON state) to spectrum II (OFF state), we find that some of the vibrational bands of 4bipy (1,011, 1,227 and 1,510 cm −1 ) broaden or shift in the ON state. Moreover, when we increased the bias voltage across the molecular junction from 10 to 800 mV, we found that one peak (1,609 cm −1 ) changed reversibly to a doublet above 100 mV ( Fig. 4b ). This splitting occurs in the nonlinear region of the current versus voltage curve (inset of Fig. 4b ). When we reversed the bias voltage, the splitting disappeared, indicating that the splitting of the peak occurs reversibly with the bias voltage. Interestingly, when we reduced the tunnelling current to 300 pA and returned the feedback to its normal setting, the chance of forming a molecular junction was significantly reduced ( Supplementary Fig. S4a ), and we did not observe splitting of the 1,609-cm −1 band ( Supplementary Fig. S4b ). This result demonstrates that the splitting of the band can only be observed at the molecular junction at a high bias voltage and that FM-TERS can reveal subtle changes in the junction that are undetectable by other methods. Figure 4: FM-TERS of 4bipy in a molecular junction and its bonding configuration. ( a ) I is an average of all 190 ON-state TERS spectra and II is a typical OFF-state TERS spectrum. Each of III, IV and V correspond to an average of ≥20 ON-state spectra. VI and VII are calculated ON- and OFF-state spectra, respectively. ( b ) The ν 8a band of 4bipy (1609 cm −1 ) is seen to change with the bias voltage (current set-point=5 nA). Inset: current versus bias curve for 4bipy obtained with a mechanical break-junction setup. ( c ) This diagram illustrates why 1,609 cm −1 band splitting is proportional to the applied bias voltage. Full size image TERS spectra in the OFF and ON states To understand these correlated spectral and molecular conductance changes, and the underlying changes in structure and bonding that occur during switching, we used cluster-model based density functional theory to qualitatively simulate TERS spectra acquired for the above states ( Supplementary Methods ). Our approach is shown schematically in Fig. 4c , and detailed in Supplementary Fig. S5 . The 4bipy molecule is composed of two pyridine rings: the one in contact with the positively biased tip is designated as the drain ring, and the one in contact with the negatively biased gold(111) substrate is the source ring. The calculated Raman spectra for the molecular junction in the ON ( Fig. 4a , spectrum VI) and OFF ( Fig. 4a , spectrum VII) states agree well with the measured spectra (I and II). In the ON state, increasing the bias voltage causes the Fermi level energy to decrease and the surface charge density on the drain electrode to increase. This leads to stronger chemical bonding between the drain electrode and the pyridine ring in contact with it. The polarizability of 4bipy increases, and Raman scattering is enhanced by an additional two or three orders of magnitude ( Supplementary Table S1 ) [34] . The significance of this additional enhancement, which occurs for the ON state but not the OFF state, is that the signal from one molecule in the ON state can be comparable with the signal from hundreds or thousands of molecules in the OFF state which are adsorbed on the substrate in the vicinity of the molecular junction. This advantage exists even when the ON-state lifetime is about a fifth of the OFF-state lifetime, as in the gold-4bipy-gold system studied here ( Fig. 3 ). It thus improves the signal-to-noise ratio achievable by FM-TERS even further, and allows the acquisition of a distinct Raman signal from the single-molecule in the junction despite the background signal from a large number of surrounding molecules which do not make contact with the tip and are therefore in the OFF state. Voltage-dependent peak splitting in the ON state can be understood in terms of the different bonding interactions which occur between the gold tip and 4bipy, and between 4bipy and the gold(111) substrate. At a low voltage, the two pyridine rings interact with the two electrodes in a similar way. As the bias voltage increases, however, the bonding interaction on the drain side will increase significantly. In our high-bias model, the gold-nitrogen bond is 2.35 Å long on the source side but only 2.15 Å long on the drain side ( Supplementary Table S2 ). The nitrogen-carbon bonds become weaker, the parallel carbon-carbon bonds become stronger, and deformation of the drain ring occurs as a result ( Supplementary Table S2 ). Therefore the frequency of the ν 8a C-N/C-C dephasing stretch increases to 1,631 cm −1 for the drain ring whereas it remains at 1,609 cm −1 for the source ring ( Supplementary Methods and Table S3 ). This is the first time that voltage-dependent changes in structure and bonding have been observed for a molecular-electronic junction, and we hope that it will invoke further study. The ability to acquire vibrational information from a molecular junction during electron transport by FM-TERS will open up new avenues of research, both experimentally and theoretically. The correlated data permits electron transport to be understood in a way that has not been possible before: by use of vibrational information obtained dominantly from the single molecule in the junction. Our FM-TERS technique is highly efficient, simple and flexible; it may soon be developed into a routine tool for this field. The ability to perform FM-TERS under ambient conditions is quite significant because these are the practical ones under which molecular electronics must function in the future. When it is combined with a Stokes/anti-Stokes capability, FM-TERS may be used to examine heating effects on the molecule forming the junction [2] , [35] , [32] . It is broadly applicable and it can be used to investigate the relationships between structure, electric properties and optical properties of various materials including graphene, quantum dots, and those used for solar energy conversion. Experimental setup of the FM-TERS instrument The setup includes a Veeco STM with an additional home-made circuit for controlling the XYZ signal and bias voltage ( Supplementary Fig. S6 , left panel). The tip current is obtained by a Digital Instruments signal access module controller and collected via 16 bit digital-to-analog and analog-to-digital cards at a very high rate of acquisition: 100,000 points s −1 to allow the plotting of reliable conductance histograms. Bias and feedback sensitivities are adjusted using Veeco software. The optical configuration of our TERS instrument is described in detail in ref. 30 , and also shown in Supplementary Fig. S6 (right panel). It consists of a home-built Raman optical fibre head, a Veeco nanoscope-E STM, and an optical fibre coupled Acton spectrometer equipped with a liquid nitrogen cooled back-illuminated CCD detector. A helium-neon laser is used to provide light with a wavelength of 632.8 nm. The beam is focused by a 50× ultralong working distance microscope objective (Olympus, numerical aperture=0.45) onto the tip-to-substrate gap with an incident angle of 60° from the surface normal in the p-polarized mode, a power of 5 mW, and a spot diameter of about 2 μm. Tip preparation Our gold tips are prepared by electrochemically etching gold wire in a mixture of fuming hydrochloric acid and anhydrous ethanol (1:1/v:v) (ref. 30 . Typically, 2 mm of a 12-mm-long straight gold wire (diameter=0.25 mm) is immersed in the etching solution at the centre of a gold wire ring (wire diameter=1 mm, ring diameter≈2 cm) placed just below the surface of the solution. The gold wire and the gold ring serve as the anode and the cathode, respectively. A potentiostat is used to fix the etching potential at 2.2 V. The electrochemical current is monitored to evaluate the quality of the tip and indicate the end of the etching process. Afterwards, the tip is rinsed thoroughly with ultrapure water (18.2 MΩ cm) or ethanol to remove etching products. A scanning electron microscope image of a typical TERS gold tip is shown in Supplementary Fig. S7 — in this case, the diameter of the apex is about 10 nm. Each tip is soaked in concentrated sulphuric acid for 15 min before use [36] . The main purpose of this step is to remove any contaminants adsorbed from the tip-etching solution or from the air afterwards. It is then soaked in ultrapure water to remove the sulphuric acid, and afterwards in ethanol to remove the water. Each tip is used for TERS immediately after drying to insure its cleanliness. Sample preparation and TERS measurement Our gold(111) single crystal substrates are prepared according to the method commonly used in surface science. The single crystal is cleaned and rinsed with piranha solution and water respectively, then annealed with a hydrogen or butane flame. The resulting single crystal is soaked in a 1 mM aqueous solution of 4bipy for 10 min. It is then rinsed with ultrapure water to remove physisorbed species and yield a clean monolayer. Finally, the electrode is blown dry with nitrogen. After the tip is in place above the gold(111) substrate at the tunnelling distance, we decrease the STM feedback setting from ~3 to ~0.001 and record the time-sequence of conductance and Raman spectra. All measurements are performed under ambient conditions, except that the whole setup is in a clean room. Theoretical methods We adopted an ion modified cluster-model based density functional theory method to simulate structure/bonding of 4bipy with gold in the OFF and ON states, and to simulate the corresponding Raman spectra ( Supplementary Methods ). A Br − Au 4 cluster was used to represent the negatively charged gold(111) substrate source electrode. The gold tip drain electrode was represented by Au 4 F − and Au 4 Cl − in two low-bias cases, and by Au 4 in a high-bias case. Thus, our model implied a static electric field pointing from the tip (+) to the substrate (−) with several appropriate bias voltages. How to cite this article: Liu, Z. et al . Revealing the molecular structure of single-molecule junctions in different conductance states by fishing-mode tip-enhanced Raman spectroscopy. Nat. Commun. 2:305 doi: 10.1038/ncomms1310 (2011).